A structural signature of liquid fragility Virtually all liquids can be maintained for some time in a supercooled state, that is, at temperatures below their equilibrium melting temperatures, before eventually crystallizing. If cooled sufficiently quickly, some of these liquids will solidify into an amorphous solid, upon passing their glass transition temperature. Studies of these supercooled liquids reveal a considerable diversity in behaviour in their dynamical properties, particularly the viscosity. Angell characterized this in terms of their kinetic fragility. Previous synchrotron X-ray scattering studies have shown an increasing degree of short- and medium-range order that develops with increased supercooling. Here we demonstrate from a study of several metallic glass-forming liquids that the rate of this structural ordering as a function of temperature correlates with the kinetic fragility of the liquid, demonstrating a structural basis for fragility. When a liquid is cooled quickly below its melting temperature, it rapidly loses kinetic energy, resulting in a sharply increasing shear viscosity and an accompanying ordering of the liquid structure. If crystallization can be avoided, the liquid eventually falls out of equilibrium and persists in a metastable amorphous state, the glass. This usually starts to occur at about 2/3 the melting temperature (liquidus) and finishes within a very narrow temperature range of only a few degrees [1] . The nature of the glass transition and why some liquids are better glass formers than others rank among the most difficult and important questions in condensed matter and materials science. First discovered more than 50 years ago [2] , metallic glasses are now finding increasing utility as novel materials for technological applications [3] . Ultimately, glass formation hinges on bypassing crystallization, which depends on a number of parameters, most notably the difference in free energy between the liquid and the solid, the interfacial free energy between the two phases and the atomic mobility, reflected in the liquid viscosity [4] . Since the viscosity varies by some 15 orders of magnitude from its value at the melting temperature to that at the glass transition temperature, it is a particularly sensitive property for characterizing different liquids. That the rate of viscosity increase with decreasing temperature varies among systems makes it a factor that is often argued to be related to glass formation, although the connection is tenuous. Angell proposed that the temperature dependences of the viscosities of different liquids can be described within the concept of fragility, described in more detail later in this article. Although generally defined in terms of dynamical properties, such as the viscosity or the relaxation rate, theoretical and experimental evidence [5] , [6] , [7] indicates that fragility is related fundamentally to thermodynamic properties, including the excess entropy and specific heat, suggesting that it should also have a structural signature. This presumed link to structural ordering is often used to qualitatively describe fragility. The results of the scattering studies presented here quantitatively confirm this connection. In the present study, high-energy synchrotron X-ray scattering studies were made on supercooled metallic glass-forming liquids in a containerless high-vacuum environment. The rate of structural ordering was determined from the rate of increase in the magnitude of the first peak in the X-ray structure factors with changing temperature. By comparing with experimental viscosity data obtained from the same liquids, also in a containerless environment, a correlation was established between the rate of structural ordering in the liquid and the fragility. Fragility is often argued to correlate with glass formability, largely because of the rate of viscosity increase over the temperature range where nucleation and growth of crystal phases are significant, as noted previously. The underlying structural basis observed here suggests that it may also be manifest in the driving and interfacial free energies. Viscosity and fragility Within the Angell concept of fragility, liquids with an approximately Arrhenius temperature dependence (nearly constant activation energy), together with a physical (phonon-like) pre-exponent, are designated as strong. As liquids show an increasing deviation from Arrhenius behaviour, they are considered to be more and more fragile. This limiting behaviour is illustrated schematically in Fig. 1 , showing the viscosities of strong and fragile liquids as a function of the inverse temperature, scaled to the glass transition temperature, T g . Ultimately, all liquids will display some non-Arrhenius behaviour at temperatures near their glass transition, but it is more dramatic for fragile liquids. Network oxides (such as SiO 2 ) are prototypical strong liquids, whereas o -terphenyl, CKN, decalin and isoquinoline are among the most fragile glass formers known. 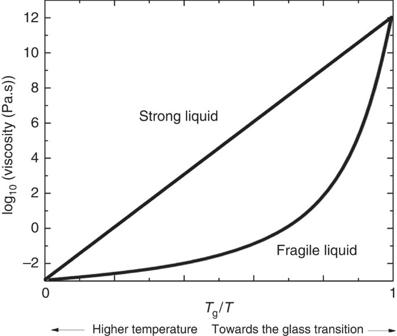Figure 1: Liquid viscosity as a function ofscaled temperature (Tg/T), illustrating Angell’s strong fragile classification. The viscosities of strong liquids have a nearly temperature-independent activation energy, while the effective activation energy for fragile (less strong) liquids dramatically increases with temperature on approaching the glass transition temperature,Tg. Figure 1: Liquid viscosity as a function of s caled temperature ( T g / T ), illustrating Angell’s strong fragile classification. The viscosities of strong liquids have a nearly temperature-independent activation energy, while the effective activation energy for fragile (less strong) liquids dramatically increases with temperature on approaching the glass transition temperature, T g . Full size image The average structure factor of liquids and glasses High-energy, wide-angle, X-ray scattering measurements were made in a transmission geometry on metallic liquids and glasses at the Advanced Photon Source (details in the Methods section). Isothermal measurements were made for several alloy liquids at temperatures ranging from several hundred degrees above to several hundred degrees below the liquidus temperature. During the measurements, the liquids were levitated in the containerless environment of the Washington University—Beamline Electrostatic Levitator [8] . Glasses were quenched for all the compositions studied, and diffraction data were obtained in a similar way to that for the liquids (details in the Methods section). While high-quality scattering data can be obtained using synchrotron sources, the interpretation of those data from amorphous samples is not straightforward. Frequently, the data are analysed using reverse Monte Carlo (RMC) methods [9] , [10] to deduce a three-dimensional structure from the one-dimensional information contained in the scattering factor. While sometimes providing a reasonable measure of the average topology of the atomic structures comprising the liquid or glass, no chemical information is obtained unless the RMC fits are constrained by other methods, such as with the results of molecular dynamics simulations. To avoid these problems, directly measured changes in the structure factor were used here to probe the structural evolution. It is somewhat surprising that the X-ray structure factors of nearly all of the metallic glass-forming liquids have a similar character, despite differences in the number of components, glass-forming ability (GFA), local atomic structure and packing, atomic size ratio [10] and extended order or networking [10] , [11] , [12] , [13] . In all metallic liquids and glasses, the first peak in the structure factor, S ( q ), sharpens and shifts to higher q with decreasing temperature, reflecting an increase in the average correlation length as well as the density, while the second peak splits or develops a shoulder, reflecting enhanced local ordering. The heights of the higher order peaks decay rapidly with q making accurate measurements of their behaviour more difficult. For illustration, the structure factors for two metallic glass-forming liquids are shown in Fig. 2 . One is Ni 62 Nb 38 , a binary alloy with rather low GFA while the other is Vit 106a, a multi-component, Zr-based five-component alloy (Zr 57 Nb 5 Cu 15.4 Ni 12.6 Al 10 ) with high GFA. Qualitatively, the structure factors for these two liquids and glasses are virtually identical. However, it is in the quantitative evolution of the structure factor with temperature that they become distinguishable. For the studies discussed here, the structure factors were measured in 12 metallic glass-forming alloys in eight distinct alloy families from high temperatures to the deeply supercooled liquid and finally the glass. The analysis was restricted to the first peak in the structure factor, S ( q 1 ), since this reflects the change of the average liquid structure, not simply the first coordination shell. In addition, since S ( q ) is essentially the normalized measured intensity, its interpretation is far less problematic than that of the structures generated from analysis methods such as RMC. It is often suggested that the pair-correlation function, the Fourier transform of the structure factor, is the measure that best represents the structure of an amorphous system. However, this function suffers from the finite- q range in the experimental data (12–15 Å −1 ), which makes it unreliable as a quantitative measure of structural evolution. 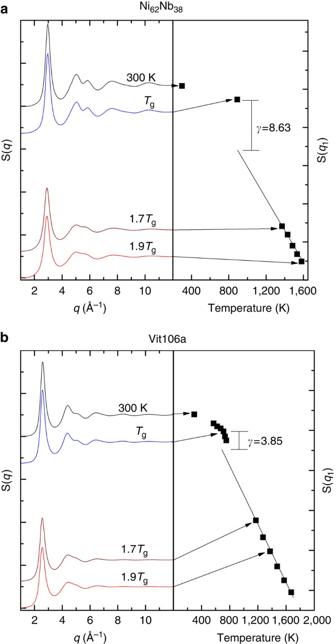Figure 2: X-ray structure factor and temperature evolution of the first peakS(q1). (a) (left) The static structure factors for Ni62Nb38are shown for the glass at room temperature (300 K) and atTg(890 K) (top) and in the liquid at two temperatures referenced toTg(bottom) (right) The height of the first peak in the structure factor,S(q1), as a function of temperature. A large discrepancy is observed between theS(q1) in the liquid when extrapolated toTgand that measured in the glass, giving a structural fragility index,γ, of 8.63. (b) The static structure factors for Vit 106a (Zr57Nb5Cu15.4Ni12.6Al10) andS(q1), shown in the same way. A much smaller discrepancy (γ=3.85) is observed, indicating more gradual ordering in the liquid to the glass structure. Figure 2: X-ray structure factor and temperature evolution of the first peak S ( q 1 ). ( a ) (left) The static structure factors for Ni 62 Nb 38 are shown for the glass at room temperature (300 K) and at T g (890 K) (top) and in the liquid at two temperatures referenced to T g (bottom) (right) The height of the first peak in the structure factor, S ( q 1 ), as a function of temperature. A large discrepancy is observed between the S ( q 1 ) in the liquid when extrapolated to T g and that measured in the glass, giving a structural fragility index, γ , of 8.63. ( b ) The static structure factors for Vit 106a (Zr 57 Nb 5 Cu 15.4 Ni 12.6 Al 10 ) and S ( q 1 ), shown in the same way. A much smaller discrepancy ( γ =3.85) is observed, indicating more gradual ordering in the liquid to the glass structure. Full size image Rapid structural evolution and a structural fragility index For illustration, the temperature dependence of the height of the first peak in S ( q ) is shown for Ni 62 Nb 38 and Vit 106a in Fig. 2a,b , respectively. Three distinct regions of behaviour are observed for Ni 62 Nb 38 : (1) the liquid, for which S ( q 1 ) evolves very slowly with temperature, dominated by changes in the local atomic structure; (2) the glass, where S ( q 1 ) also changes slowly but owing to atomic vibrational contributions rather than significant structural rearrangements; and (3) an experimentally inaccessible region linking the other two regions that requires an acceleration in the development of S ( q 1 ). This acceleration of order has been observed in a few metallic glass-forming systems with poor GFA [14] , [15] , [16] and this behaviour is contrasted with that of the evolution of S ( q 1 ) for Vit 106a, where it changes gradually from the liquid to the glass ( Fig. 2b ). Essentially, no accelerated evolution occurs in the intermediate region for Vit 106a, a behaviour that has been previously presented for a few bulk metallic glass-forming alloys, but not analysed in this manner [17] , [18] , [19] . The very different behaviours of Ni 62 Nb 38 and Vit 106a are analogous to the fragile/strong characterization of viscosity proposed by Angell. However, while Angell’s fragility reflects a characterization of a kinetic measurement, these results point to an underlying structural signature. We define a structural fragility index, γ , as the mismatch between the value for S ( q 1 ) in the liquid when extrapolated to T g and the value measured in the glass at that temperature, that is, Like the common fragility index m , γ increases with the fragility of the liquid. Measurements of viscosity and liquid fragility To make a more quantitative comparison between the kinetic and structural aspects of fragility, the liquid viscosity was measured at high temperatures in the containerless environment of the electrostatic levitation (ESL) (see Methods section). The viscosities of all of the liquids measured are shown in Fig. 3a , with inverse temperature scaled to the experimentally measured calorimetric glass transition temperatures. At any temperature, T , the activation energy is proportional to the local slope, dlog( η )/d( T g / T ), where η is the viscosity. While small for all metallic liquids, the value of the activation energy at high temperatures increases with the strength of that liquid. For strong liquids, the activation energy increases modestly upon approaching T g , while fragile liquids show a much larger increase. The data in Fig. 3a show that the magnitude of the viscosity also increases with the strength of the liquid, with stronger liquids located towards the top of the plot and more fragile ones located at the bottom. The correlation between the magnitudes of the viscosities and the values of the activation energies at high temperatures, far away from T g, for all liquids studied is shown in Fig. 3b . Although shown only for a specific value of T g / T (0.55), the correlation holds well over the measured temperature range studied (0.5≤ T g /T ≤0.6). 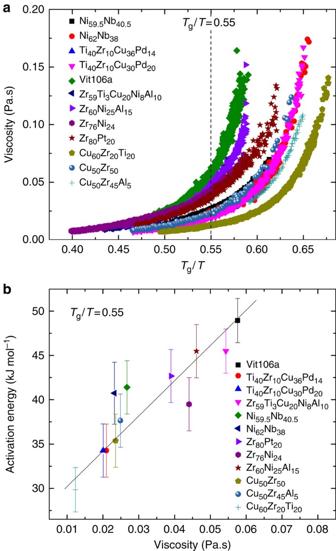Figure 3: Measured magnitude and activation energy of viscosity for all liquids studied. (a) The viscosity as a function of reduced temperature for the liquid compositions listed in the legend. (b) The correlation between the activation energy and the viscosity calculated from the data inFig. 3aat a reduced temperature ofTg/T=0.55. A strong correlation emerges at all reduced temperatures for which data are available. Figure 3: Measured magnitude and activation energy of viscosity for all liquids studied. ( a ) The viscosity as a function of reduced temperature for the liquid compositions listed in the legend. ( b ) The correlation between the activation energy and the viscosity calculated from the data in Fig. 3a at a reduced temperature of T g / T =0.55. A strong correlation emerges at all reduced temperatures for which data are available. Full size image The degree to which the viscosity displays non-Arrhenius behaviour is often parameterized by fits to the Vogel–Fulcher–Tammann (VFT) equation, where η 0 is the viscosity in the infinite temperature limit and T 0 is the temperature at which the viscosity becomes infinite. The quantity D * is a measure of the fragility of the liquid, called the kinetic strength to differentiate it from the fragility index, which is defined near T g . As D * increases, the behaviour of the VFT equation becomes more Arrhenius-like, consistent with a stronger (less fragile) liquid [20] . Since the viscosity data were obtained at high temperatures, D * is the more appropriate parameter for assessing the fragility of the liquids in Fig. 3 , rather than m . Structural fragility The structural fragility index correlates well with the fragility behaviour obtained from the viscosity data in Fig. 3 , in terms of both the local activation energy ( Fig. 4a ) and the kinetic strength ( Fig. 4b ). For Fig. 4b , D * was determined by fitting equation (2) to the experimental data, assuming that the viscosity is equal to 10 12 Pa.s at the calorimetric glass transition. It should be pointed out that another common practice for obtaining D * is to set T 0 equal to the glass transition temperature, since the two are close for many metallic liquids [20] , [21] . While this approach produces systematically lower values for D *, the correlation with the structural fragility index found in Fig. 4b is unchanged. 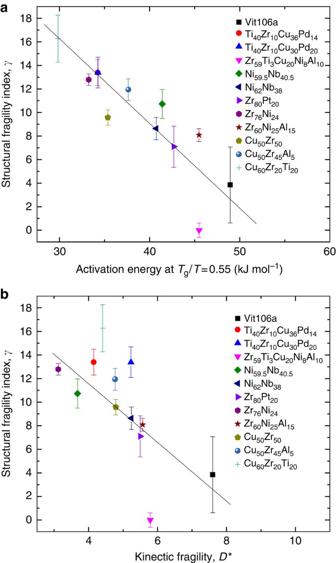Figure 4: Correlation between structural fragility and kinetic fragility. The structural structural fragility index shown (a) as a function of the activation energy of the shear viscosity atTg/T=0.55 and (b) as a function of the kinetic strength,D*. Figure 4: Correlation between structural fragility and kinetic fragility. The structural structural fragility index shown ( a ) as a function of the activation energy of the shear viscosity at T g / T =0.55 and ( b ) as a function of the kinetic strength, D *. Full size image A structural fragility parameter based on the temperature dependence of the width of the first peak in S ( q ) has been previously suggested [22] . However, as shown in Fig. 5 , the correlation between either the temperature-dependent peak width or the position of the first peak in S ( q ) and the kinetic fragility is significantly poorer than with the peak height. The structural fragility index, γ , was defined in equation (1) as the mismatch between the value for S ( q 1 ) in the liquid when extrapolated to T g and the value measured in the glass at that temperature. Analogous measures to the mismatch in the first peak position in S ( q ), were also computed for q 1 , ( Fig. 5a ) and the width of the first peak in S ( q ) (at half maximum) ( Fig. 5b ). Unlike the structural fragility, the correlation between the mismatch of these quantities and the kinetic fragility is extremely poor. Changes in the profile of the first peak in S ( q ) are correlated with ordering in the liquid. The lack of a strong correlation between changes in the peak width and the fragility likely arises from a difficulty to accurately resolve the small changes with temperature. The changes in the peak height are larger and more easily measured. Further, it should be noted that other related quantities, such as the sound velocity [23] , [24] , and the results from light scattering [25] and inelastic X-ray scattering studies [26] , have been related to the liquid fragility and to sudden structural changes near T g in more complex liquid families. When taken with the direct structural measurements reported here, the conclusion of a deep connection between structure and dynamics in supercooled liquids and glasses is broadly supported. 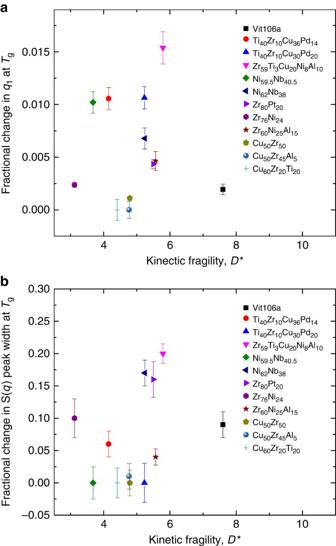Figure 5: Correlation betweenS(q) peak position and peak width and kinetic fragility. The correlation between the temperature-dependent peak position (Fig. 5a) or the full width at half maximum of the first peak inS(q) (Fig. 5b) and the kinetic fragility is significantly poorer than with the peak height shown inFig. 4b. Figure 5: Correlation between S ( q ) peak position and peak width and kinetic fragility. The correlation between the temperature-dependent peak position ( Fig. 5a ) or the full width at half maximum of the first peak in S ( q ) ( Fig. 5b ) and the kinetic fragility is significantly poorer than with the peak height shown in Fig. 4b . Full size image It is tempting to correlate fragility with GFA. It has been argued, for example, that strong liquids tend to have a higher GFA than fragile ones [27] , [28] , [29] , [30] and that those metallic liquids containing more components are generally stronger and have a higher GFA than liquids with fewer components [30] . Since the data presented here demonstrate that fragility reflects the rate of structural ordering near T g , connections can be made to the results of molecular dynamics investigations of GFA. Studies of Cu–Zr liquids and glasses [11] , [31] , [32] , [33] indicate that the development of ordered clusters in the supercooled liquid, which form a backbone of connected clusters that grows rapidly near T g , are distinguishing features of the best glass-forming compositions in this alloy. Theoretical studies show that the rate of dominant local ordering (icosahedral, in these cases) in fragile liquids is accelerated near the glass transition temperature [11] , [31] , [32] , [34] . It is unlikely that all liquids will show strong icosahedral ordering; the order in Zr–Ni and Ni–Nb liquids, for example, is likely fundamentally different from the icosahedral order in Cu–Zr liquids [10] , [35] . So, it is the rate of ordering in the liquid near T g and the similarity in the local atomic ordering between the liquid and the glass, not the type of ordering, that underlay fragility. Further, it is important to emphasize that while frequently invoked, the link between GFA and kinetic fragility is a rather weak correlation that often fails [36] , [37] ; other factors that are not described by fragility, such as heterogeneous nucleation, can be critical. In conclusion, the combined structural and viscosity data presented here demonstrate the connection between kinetic fragility and liquid structure. A structural parameter, γ , can be introduced to characterize the liquid fragility, correlated with the rate of structural ordering with decreasing temperature. While icosahedral ordering is dominant in many liquids, γ is not tied to the specific type of local order, making it potentially a universal parameter. The often-quoted link between fragility and glass-forming ability arises from the coupling of fragility with structure and dynamics, determining the viscosity and the driving and interfacial free energies for crystallization. Of most interest, however, is that the results presented here clearly show a fundamental link between structure and dynamics. Sample preparation Samples were prepared from ~1 g master-ingots made using high-purity raw materials by arc-melting on a water-cooled Cu hearth in a high-purity Ar gas atmosphere (99.998%). The arc-melting chamber was repeatedly evacuated to less than 50 mtorr and backfilled with Ar. A Ti–Zr getter, located near the sample ingots, was kept molten for about 1 min to further reduce residual oxygen before melting the samples. Each ingot was melted three times to ensure a homogeneous composition; the ingot was discarded in case the mass loss exceeded 0.05%. The ESL samples (60–90 mg) were made from portions of the master ingot by a single arc-melting. Metallic glass ribbons were prepared by melting portions of the master ingot in a graphite crucible using radio frequency induction heating, and rapidly quenching the high-temperature liquid onto a rotating copper wheel, producing quenching rates ~10 5 –10 6 K s −1 . ESL The ESL technique was used to prepare metallic liquids in the equilibrium and supercooled liquid state. By levitating the sample in vacuum (~10 −7 Torr) heterogeneous nucleation, catalysed by contact with air and/or the container, is avoided, allowing data to be acquired from the supercooled liquid. The temperature was measured using a Metis MQ22 two-color ratio pyrometer (Process Sensors), operating at 1.40 and 1.64 μm wavelengths. Details of the ESL, including how samples are levitated and thermally processed and how the ESL is interfaced with high-energy X-ray beamlines, are provided elsewhere [8] . Structural measurements High-energy X-ray diffraction data for both the liquids and the glasses were obtained at the advanced photon source on beamline 6-ID-D. For the glass measurements, the samples were placed in capillary tubes having wall thicknesses of 10 μm. The tubes were evacuated to reduce oxidation and were placed in a custom-built furnace to heat the ribbons to temperatures up to and above the glass transition temperature. The effective Debye temperatures and structural relaxation effects in the glasses were determined from the temperature evolution of the structure factors during thermal cycling. High-energy diffraction measurements of the liquids and glasses ( E =129 keV, λ =0.0969 Å −1 for the liquid studies and E =100 keV, λ =0.1243 Å −1 for the glass studies) were made in a transmission geometry to a momentum transfer, q , of 15 Å −1 using a GE Revolution 41-RT amorphous Si flat-panel X-ray detector. The static structure factor, S ( q ), was derived from the scattering data by first applying an appropriate gain map, masking bad pixels, averaging images, subtracting the appropriate background and correcting for oblique incidence, absorption, sample geometry, multiple scattering, fluorescence, Compton scattering and secondary container-scattering contributions using in-house analysis packages written in LabView. [38] Diffraction data for the liquids were obtained as a function of temperature by interfacing the electrostatic levitator with the beamline. Scattering data were collected in a series of isothermal holds over a wide temperature range; the duration of the holds were 20 s for all samples. Viscosity measurements The viscosity at each temperature was measured using the oscillating drop technique [39] , [40] , in which the levitation electric field was modulated near the l =2 (second spherical harmonic, or surface dipole oscillation) resonant frequency (120–140 Hz) of the liquid to induce surface vibrations. The surface deformation was captured as high-speed (1,560 frames per second) videos of the silhouettes of the liquid samples. Intensity summation of each video frame varied in proportion to the amplitude of the second harmonic oscillation. After the perturbation was removed, the amplitude of the surface harmonic oscillations damped exponentially, with a time constant inversely proportional to the viscosity [41] . The kinetic strength, D *, was determined for each liquid by fitting the high-temperature viscosity data to the VFT formula. The viscosity at the glass transition temperature was set to 10 12 Pa.s. In all cases, the fit VFT temperatures ( T 0 ) were on the order of 100 K below the calorimetric glass transition temperature, consistent with previous findings [42] , [43] , [44] . How to cite this article: Mauro, N. A. et al. A structural signature of liquid fragility. Nat. Commun. 5:4616 doi: 10.1038/ncomms5616 (2014).